Hepatoprotective role of Sestrin2 against chronic ER stress Upon prolonged endoplasmic reticulum (ER) stress, cells attenuate protein translation to prevent accumulation of unfolded proteins. Here we show that Sestrin2 is critical for this process. Sestrin2 expression is induced by an ER stress-activated transcription factor CCAAT-enhancer-binding protein beta (c/EBPβ). Once induced, Sestrin2 halts protein synthesis by inhibiting mammalian target of rapamycin complex 1 (mTORC1). As Sestrin2-deficient cells continue to translate a large amount of proteins during ER stress, they are highly susceptible to ER stress-associated cell death. Accordingly, dietary or genetically induced obesity, which does not lead to any pathological indication other than simple fat accumulation in the liver of wild-type (WT) mice, can provoke Sestrin2-deficient mice to develop severe ER stress-associated liver pathologies such as extensive liver damage, steatohepatitis and fibrosis. These pathologies are suppressed by liver-specific Sestrin2 reconstitution, mTORC1 inhibition or chemical chaperone administration. The Sestrin2-mediated unfolded protein response (UPR) may be a general protective mechanism against ER stress-associated diseases. Excessive hepatic fat accumulation during obesity and non-alcoholic fatty liver disease (NAFLD) can induce chronic endoplasmic reticulum (ER) stress, a perturbation in ER homeostasis that can lead to hepatocyte death and a subsequent series of liver inflammation, oxidative stress accumulation and fibrosis collectively known as non-alcoholic steatohepatitis (NASH) [1] , [2] . However, the progression from simple hepatosteatosis to NASH does not occur rapidly in most experimental models and human clinical cases of obesity. For example, although overnutrition in rodents, caused by high-fat diet (HFD) feeding or leptin deficiency, can result in obesity and hepatosteatosis, it does not spontaneously provoke steatohepatitis or fibrosis without further liver injury [3] , [4] . In humans, a substantial portion of the population with obesity and hepatosteatosis shows fairly stable NAFLD symptoms for a prolonged period without progressing to NASH [5] . This attenuation of NASH development can be due to the existence of protective mechanisms that suppress obesity-associated ER stress. A mechanism that protects cells against ER stress is generally defined as unfolded protein response (UPR) [6] . Perturbation of ER homeostasis leads to activation of three transmembrane ER stress sensor molecules: protein kinase RNA-like ER kinase (PERK), inositol-requiring enzyme 1 (IRE1) and activating transcription factor 6 (ATF6). These ER stress sensors together initiate protective UPR that increases molecular chaperone levels, attenuates protein synthesis and ER protein loading and upregulates ER-associated protein degradation and ER membrane biosynthesis. However, persistent and robust ER stress that exceeds the capacity of protective UPR may lead to cell death through apoptotic signalling activation [7] or ATP depletion [8] . The failure in protective UPR and the subsequent induction of ER stress-induced cell death are detrimental to physiological homeostasis, and these damages have been implicated in diverse degenerative diseases associated with obesity [9] . However, the detailed molecular mechanisms underlying the protective UPR have not been completely understood yet. Sestrins are a family of stress-inducible proteins that can suppress mammalian target of rapamycin complex 1 (mTORC1) through activation of AMP-activated protein kinase (AMPK) [10] , [11] . Sestrins are necessary for maintaining metabolic homeostasis and preventing age- and obesity-associated pathologies [11] , [12] , [13] . Among the three Sestrin homologues in mammals (Sestrin1–3), we recently found that, through unknown mechanisms, Sestrin2 expression in the liver becomes elevated upon hypernutrition and obesity and functions to alleviate insulin resistance and hepatosteatosis [12] . Here we show that Sestrin2 is transcriptionally induced through the PERK–c/EBPβ (CCAAT-enhancer-binding protein beta) pathway upon obesity-associated ER stress and maintains hepatic ER homeostasis by suppressing mTORC1-dependent protein translation. Correspondingly, loss of Sesn2 allows for persistent protein synthesis in hepatocytes even under chronic ER stress, which further exacerbates the level of ER stress and subsequently results in extensive NASH-like pathologies such as liver damage, inflammation and fibrosis. Our results suggest that Sestrin2 critically mediates hepatocellular adaptation to ER stress and that Sestrin2 is the endogenous attenuator of NAFLD progression that operates primarily through maintaining ER homeostasis. Induction of Sestrin2 expression by ER stress insults To understand how Sestrin2 expression is induced upon obesity, we subjected the human HepG2 cells to a series of culture environments that could mimic the conditions during obesity. As a result, we found that saturated fatty acids (SFAs) such as palmitic acid (PA) or stearic acid induced prominent accumulation of Sestrin2 mRNA and protein ( Fig. 1a–c and Supplementary Fig. 1a ). In contrast, unsaturated fatty acids such as oleic acid or docosahexaenoic acid not only failed to induce this upregulation ( Supplementary Fig. 1b,c ) but actually suppressed the effect of SFA ( Supplementary Fig. 1d,e ). Interestingly, the patterns of Sestrin2 expression were almost entirely correlated with the patterns of ER stress signalling activation that was monitored by PERK phosphorylation, c/EBP homologous protein (CHOP) expression and X-box binding protein 1 (XBP1) splicing ( Fig. 1a and Supplementary Fig. 1a–e ). Chemical ER stress inducers such as tunicamycin (Tm) or thapsigargin also induced Sestrin2 expression in HepG2 cells ( Supplementary Fig. 1f,g ) and mouse liver ( Supplementary Fig. 1h ). 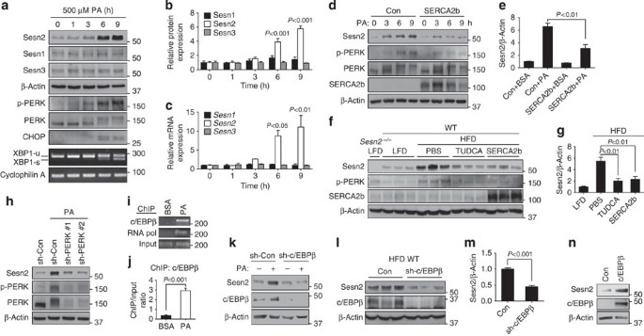Figure 1: Obesity induces Sestrin2 through ER stress signalling. (a–c) HepG2 cells were treated with PA for indicated hours and analysed by immunoblotting (images with black bands) and RT–PCR (images with white bands).Pvalues were calculated between untreated (0 h) and indicated groups (b,c;n=3). (d,e) At 48 h after infection with green fluorescent protein (GFP; Con)- or SERCA2b-overexpressing adenoviruses, cells were treated with BSA (0 h) or PA for indicated hours (d) or 9 h (e;n=3). (f,g,l,m) Six-month-old WT mice kept on low-fat diet (LFD) or HFD for 4 months were injected daily with vehicle (phosphate-buffered saline (PBS)) or TUDCA (500 mg per kg body weight i.p.) or transduced once with adenoviruses expressing SERCA2b, GFP (Con) or shRNA targeting c/EBPβ. After 10 days, livers were analysed by immunoblotting (n=3). (h,k) At 48 h before PA treatment, cells were infected with lentiviruses expressing shRNAs targeting luciferase (Con), PERK (h) and c/EBPβ (k). After 9 h of BSA (−) or PA treatment, cells were analysed by immunoblotting. (i,j) ChIP analysis of cells with indicated treatments (n=3). (n) At 24 h after infection with GFP (Con)- or c/EBPβ-overexpressing adenoviruses, cells were analysed by immunoblotting. All data are shown as the mean±s.e.m.Pvalues are from Student’st-test. Molecular weight markers are indicated in kDa (immunoblots) or bp (agarose gels). Figure 1: Obesity induces Sestrin2 through ER stress signalling. ( a – c ) HepG2 cells were treated with PA for indicated hours and analysed by immunoblotting (images with black bands) and RT–PCR (images with white bands). P values were calculated between untreated (0 h) and indicated groups ( b , c ; n =3). ( d , e ) At 48 h after infection with green fluorescent protein (GFP; Con)- or SERCA2b-overexpressing adenoviruses, cells were treated with BSA (0 h) or PA for indicated hours ( d ) or 9 h ( e ; n =3). ( f , g , l , m ) Six-month-old WT mice kept on low-fat diet (LFD) or HFD for 4 months were injected daily with vehicle (phosphate-buffered saline (PBS)) or TUDCA (500 mg per kg body weight i.p.) or transduced once with adenoviruses expressing SERCA2b, GFP (Con) or shRNA targeting c/EBPβ. After 10 days, livers were analysed by immunoblotting ( n =3). ( h , k ) At 48 h before PA treatment, cells were infected with lentiviruses expressing shRNAs targeting luciferase (Con), PERK ( h ) and c/EBPβ ( k ). After 9 h of BSA (−) or PA treatment, cells were analysed by immunoblotting. ( i , j ) ChIP analysis of cells with indicated treatments ( n =3). ( n ) At 24 h after infection with GFP (Con)- or c/EBPβ-overexpressing adenoviruses, cells were analysed by immunoblotting. All data are shown as the mean±s.e.m. P values are from Student’s t -test. Molecular weight markers are indicated in kDa (immunoblots) or bp (agarose gels). Full size image Obesity induces Sestrin2 through ER stress signalling Overexpression of sarco-ER calcium pump 2b (SERCA2b) or administration of a chemical chaperone tauroursodeoxycholic acid (TUDCA), either of which can substantially reduce hepatic ER stress [14] , [15] , [16] , was able to halt Sestrin2 induction caused by SFA ( Fig. 1d,e ; in HepG2 cells) or HFD-induced obesity ( Fig. 1f,g and Supplementary Fig. 1i–k ; in mouse liver). On the contrary, other known regulators of the Sestrin-family gene expression, such as oxidative stress, c-Jun N-terminal kinase (JNK), p53 or mTORC1, were not involved in Sestrin2 induction during obesity; antioxidants, SP600125, p53-shRNA (p53-short-hairpin RNA) and rapamycin failed to suppress SFA- or obesity-induced Sestrin2 expression ( Supplementary Fig. 1l–x ). Thus, we concluded that obesity increases Sestrin2 expression primarily through activation of ER stress signalling. PERK–c/EBPβ axis mediates Sestrin2 induction upon ER stress We next searched for a molecular mechanism by which the ER stress signal could be sensed and transmitted to induce Sestrin2 expression upon obesity. Inhibition of an ER stress sensor PERK, but not that of the other two sensors IRE1 and ATF6, abolished the ability of SFA to induce Sestrin2 ( Fig. 1h and Supplementary Fig. 2a,b ). ATF4 and CHOP, the two most well-characterized transcription factors downstream of PERK [6] , were not involved in SFA-induced Sestrin2 expression ( Supplementary Fig. 2c,d ), whereas c/EBPβ, another transcription factor downstream of PERK [17] , [18] whose active isoform (LAP) accumulates inside the nucleus ( Supplementary Fig. 2e,f ) and binds to the Sesn2 promoter upon ER stress insults ( Fig. 1i,j and Supplementary Fig. 2g,h ), was both necessary and sufficient to induce SFA- or obesity-induced Sestrin2 expression ( Fig. 1k–n ). These results indicate that the PERK–c/EBPβ signalling pathway controls Sestrin2 expression during obesity-associated ER stress. Sestrin2 links ER stress and AMPK-mTORC1 regulation Several recent studies indicate that chronic ER stress suppresses mTORC1 through an unknown mechanism that involves the activation of PERK and AMPK [19] , [20] . Our findings here regarding the ER stress-induced Sestrin2 expression suggest that Sestrin2 may be the unknown moderator that bridges ER stress signalling and mTORC1 function. Indeed, Sestrin2-deficient cells and tissues could not activate AMPK or inhibit mTORC1 signalling upon SFA- ( Fig. 2a–e ) or Tm-induced ER stress ( Fig. 2f–h ). The signalling misregulation was not due to defects in energy homeostasis as cellular ATP levels were not significantly altered by either Sestrin2 deficiency or ER stress insults ( Fig. 2i,j ). These results demonstrate that mTORC1 suppression during ER stress is dependent on Sestrin2. 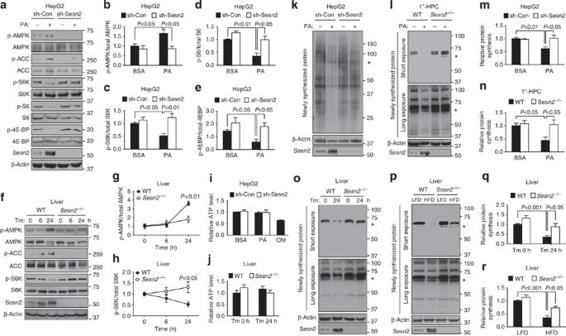Figure 2: Sestrin2 suppresses mTORC1 and protein synthesis in response to ER stress. (a–e) At 48 h after infection with shRNA lentiviruses for luciferase (Con) or Sestrin2, HepG2 cells were treated with PA for 9 h and analysed by immunoblotting (n=3). AMPK signalling activity was monitored by phosphorylation of AMPK and acetyl-CoA carboxylase (ACC). mTORC1 signalling activity was monitored by phosphorylation of p70 ribosomal S6K, ribosomal protein S6 and eIF4E-binding protein (4E-BP). (f–h) Two-month-old WT orSesn2−/−mice kept on LFD were injected with Tm (500 mg per kg body weight i.p.). After indicated hours, livers were analysed by immunoblotting (n=4). (i,j) Relative intracellular ATP levels of indicated cells (i,n=3) and liver tissues (j,n=4). As a positive control for ATP depletion, HepG2 cells were treated with oligomycin (OM, 5 μg ml−1) for 1 h. (k–r) HepG2 cells transduced with sh-Con or sh-Sesn2 (k,m,n=5) or primary hepatocytes (1°-HPC) isolated from WT orSesn2−/−mice (l,n,n=4) were treated with BSA (−) or PA for 9 h. Two-month-old WT orSesn2−/−mice were injected with Tm (o,q,n=4) or kept on LFD or HFD for additional 2 months (p,r,n=4). After indicated treatments, newly synthesized proteins in cells (k–n) and liver tissues (o–r) were visualized and quantified using the Click-IT AHA labelling system. The protein bands denoted by stars correspond to serum albumin (70 kD), which is the most actively synthesized protein in normal hepatocytes. All data are shown as the mean±s.e.m.Pvalues are from Student’st-test. Molecular weight markers are indicated in kDa. Figure 2: Sestrin2 suppresses mTORC1 and protein synthesis in response to ER stress. ( a – e ) At 48 h after infection with shRNA lentiviruses for luciferase (Con) or Sestrin2, HepG2 cells were treated with PA for 9 h and analysed by immunoblotting ( n =3). AMPK signalling activity was monitored by phosphorylation of AMPK and acetyl-CoA carboxylase (ACC). mTORC1 signalling activity was monitored by phosphorylation of p70 ribosomal S6K, ribosomal protein S6 and eIF4E-binding protein (4E-BP). ( f – h ) Two-month-old WT or Sesn2 −/− mice kept on LFD were injected with Tm (500 mg per kg body weight i.p.). After indicated hours, livers were analysed by immunoblotting ( n =4). ( i , j ) Relative intracellular ATP levels of indicated cells ( i , n =3) and liver tissues ( j , n =4). As a positive control for ATP depletion, HepG2 cells were treated with oligomycin (OM, 5 μg ml −1 ) for 1 h. ( k – r ) HepG2 cells transduced with sh-Con or sh-Sesn2 ( k , m , n =5) or primary hepatocytes (1°-HPC) isolated from WT or Sesn2 −/− mice ( l , n , n =4) were treated with BSA (−) or PA for 9 h. Two-month-old WT or Sesn2 −/− mice were injected with Tm ( o , q , n =4) or kept on LFD or HFD for additional 2 months ( p , r , n =4). After indicated treatments, newly synthesized proteins in cells ( k – n ) and liver tissues ( o – r ) were visualized and quantified using the Click-IT AHA labelling system. The protein bands denoted by stars correspond to serum albumin (70 kD), which is the most actively synthesized protein in normal hepatocytes. All data are shown as the mean±s.e.m. P values are from Student’s t -test. Molecular weight markers are indicated in kDa. Full size image Sestrin2 attenuates translation during chronic ER stress Although PERK-mediated eukaryotic translation initiation factor 2α (eIF2α) phosphorylation can halt protein translation during the early phase of ER stress, this inhibitory effect is only temporary and quickly diminished during prolonged ER stress [6] , [8] . Paradoxically, other ER stress signalling components downstream of PERK and eIF2α, such as ATF4 and CHOP, were found to increase protein synthesis and antagonize the effect of eIF2α phosphorylation [8] . Considering that mTORC1 is a major regulator of protein translation, Sestrin2-mediated mTORC1 suppression that occurs during ER stress may provide an alternative explanation for the inhibition of protein translation. During the early phase of ER stress (within 3 h of SFA treatment), Sestrin2-deficient cells properly ceased protein translation similarly to control cells ( Supplementary Fig. 3a,b ). However, after 9 h of SFA-induced ER stress, Sestrin2-deficient HepG2 cells and mouse primary hepatocytes continued to translate large amounts of proteins, while control cells managed to cease protein synthesis under the same condition ( Fig. 2k–n and Supplementary Fig. 3a–c ), suggesting that Sestrin2 is indeed critical for protein synthesis regulation during chronic ER stress. Similarly, Sesn2 −/− mice could not downregulate hepatic protein synthesis upon 24 h of Tm treatment or 2 months of HFD feeding ( Fig. 2o–r and Supplementary Fig. 3d–g ) in contrast to wild-type (WT) mice [8] , [15] . On the other hand, mTORC1 inhibition by Sestrin2 overexpression or rapamycin treatment was sufficient to suppress protein translation ( Supplementary Fig. 3h,i ) without inducing eIF2α phosphorylation or ATF4 expression ( Supplementary Fig. 3j,k ). Therefore, Sestrin2 is a critical mediator of UPR that halts mTORC1-dependent protein translation during chronic ER stress. Sestrin2 deficiency aggravates ER stress during obesity Cessation of protein translation is critical for decreasing ER protein load and preventing accumulation of unfolded proteins. Thus, we were curious whether Sestrin2 was necessary for resolution of ER stress after insults. Sestrin2 deficiency strongly exacerbated SFA-induced ER stress in HepG2 cells and mouse primary hepatocytes, as evidenced by increased phosphorylation of PERK and eIF2α and upregulation of ER stress-induced gene expression ( Supplementary Fig. 4a–d ). Sesn2 −/− mice also exhibited extensive aggravation of ER stress, either upon Tm treatment- ( Fig. 3a,b and Supplementary Fig. 4e–g ), HFD- ( Fig. 3c–f and Supplementary Fig. 4h,i ) or Lep ob mutation-induced obesity ( Fig. 3g–i and Supplementary Fig. 4j ). Hyperactivated ER stress signalling in obese Sesn2 −/− mouse liver was completely suppressed by liver-specific transduction of Sestrin2 ( Supplementary Fig. 5a–d ), suggesting that Sestrin2 suppresses hepatic ER stress in a tissue-autonomous manner. 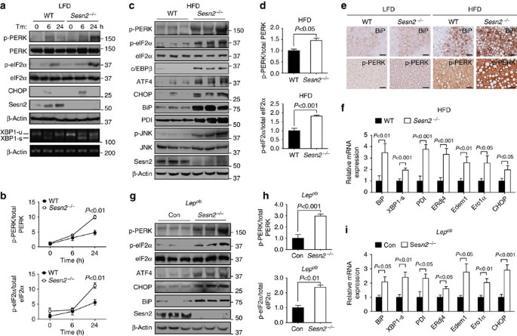Figure 3: Sestrin2 deficiency exacerbates ER stress upon chemical insults or obesity. (a,b) Two-month-old WT orSesn2−/−mice kept on LFD were injected with Tm (500 mg per kg body weight, i.p.). After indicated hours, livers were harvested from the treated mice and analysed (n=4). Protein phosphorylation and expression were analysed by immunoblotting (images with black bands) (a) and quantified (b). XBP1 mRNA splicing was examined through semi-quantitative RT–PCR (images with white bands) (a). (c–i) Six-month-old WT (n=6) andSesn2−/−(n=5) mice kept on LFD or HFD for 4 months (c–f) and 4-month-oldLepob/ob/Sesn2+/−(Con,n=4) andLepob/ob/Sesn2−/−(n=6) mice kept on LFD (g–i) were analysed. Protein phosphorylation and expression were analysed by immunoblotting (c,g) and quantified by densitometry (d,h). Liver sections were stained with indicated antibodies (e). Relative mRNA expression of ER stress-inducible genes was quantified through qRT–PCR (f,i). Scale bars, 100 μm. All data are shown as the mean±s.e.m.Pvalues are from Student’st-test. Molecular weight markers are indicated in kDa (immunoblots) or bp (agarose gels). Figure 3: Sestrin2 deficiency exacerbates ER stress upon chemical insults or obesity. ( a , b ) Two-month-old WT or Sesn2 −/− mice kept on LFD were injected with Tm (500 mg per kg body weight, i.p.). After indicated hours, livers were harvested from the treated mice and analysed ( n =4). Protein phosphorylation and expression were analysed by immunoblotting (images with black bands) ( a ) and quantified ( b ). XBP1 mRNA splicing was examined through semi-quantitative RT–PCR (images with white bands) ( a ). ( c – i ) Six-month-old WT ( n =6) and Sesn2 −/− ( n =5) mice kept on LFD or HFD for 4 months ( c – f ) and 4-month-old Lep ob/ob / Sesn2 +/− (Con, n =4) and Lep ob/ob / Sesn2 −/− ( n =6) mice kept on LFD ( g – i ) were analysed. Protein phosphorylation and expression were analysed by immunoblotting ( c , g ) and quantified by densitometry ( d , h ). Liver sections were stained with indicated antibodies ( e ). Relative mRNA expression of ER stress-inducible genes was quantified through qRT–PCR ( f , i ). Scale bars, 100 μm. All data are shown as the mean±s.e.m. P values are from Student’s t -test. Molecular weight markers are indicated in kDa (immunoblots) or bp (agarose gels). Full size image Sestrin2 controls ER homeostasis through AMPK-mTORC1 Sestrin2 has two independent biological activities largely divided into regulating the AMPK-mTORC1 signalling and suppressing the reactive oxygen species (ROS) accumulation [11] . We found that, in Sestrin2-silenced cells, ER stress was strongly reduced by aminoimidazole carboxamide ribonucleotide (AICAR, an activator of AMPK) and rapamycin as well as by another mTORC1 inhibitor PP242 and a translation inhibitor cycloheximide ( Fig. 4a–c and Supplementary Fig. 6a,b ), while treatment of antioxidants such as BHA and N-acetylcysteine turned out to be ineffective ( Fig. 4b,c ). Inhibition of mTORC1 by Raptor-shRNA also ameliorated excessive ER stress signalling in Sestrin2-deficient cells ( Fig. 4d,e ), while mTORC1 activation by TSC2-shRNA exacerbated PA-induced ER stress ( Fig. 4f,g ). In liver of obese Sesn2 −/− mice, liver-specific AMPK CA transduction or systemic AICAR administration was sufficient to suppress ER stress signalling ( Fig. 4h–k and Supplementary Fig. 6c,d ). Consistent with the known roles of mTORC1 in regulating protein translation, AICAR, rapamycin and cycloheximide all suppressed protein translation in SFA-treated Sestrin2-deficient cells ( Supplementary Fig. 6e,f ), whereas TSC2 inhibition upregulated protein synthesis in SFA-treated control cells ( Supplementary Fig. 6g,h ). We also tested whether alleviation of protein synthesis through the eIF2a pathway could reduce ER stress in Sesn2 −/− mice. Salubrinal, a specific inhibitor of eIF2α dephosphorylation [21] ( Supplementary Fig. 7a,b ), substantially suppressed ER stress in livers of Sesn2 −/− mice ( Supplementary Fig. 7c–e ). Taken together, our findings indicate that Sestrin2 maintains ER homeostasis primarily through regulation of the AMPK-mTORC1-protein synthesis signalling pathway. 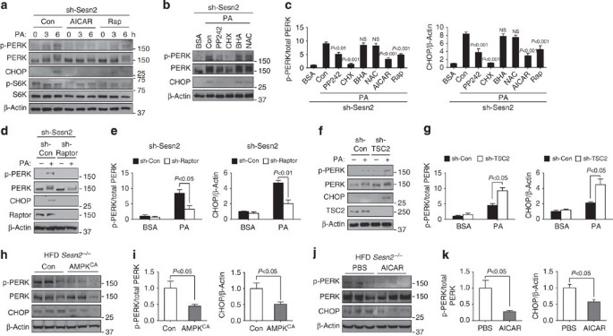Figure 4: Sestrin2 controls ER homeostasis through the AMPK-mTORC1 axis. (a–c) HepG2 cells stably transduced with Sestrin2 shRNA (sh-Sesn2) were treated with PA for indicated hours (a) or 6 h (b). PBS (Con), AICAR (1 mM), Rapamycin (Rap, 100 nM), PP242 (1 μM), cycloheximide (CHX, 180 μM), BHA (100 μM) and NAC (10 mM) were applied 1 h before treating with PA. AICAR is an AMPK activator, PP242 is an mTOR inhibitor and CHX is a protein translation inhibitor. Protein phosphorylation and expression were examined (a,b) and quantified (c) (n=3).Pvalues were calculated between PA+PBS (Con) and indicated groups. (d,e) Sestrin2-silenced HepG2 cells were transduced with shRNA lentiviruses for luciferase (Con) or Raptor (sh-Raptor). After 48 h, cells were treated with BSA (−) or PA for 6 h and analysed by immunoblotting (n=3). (f,g) At 48 h after infection with shRNA lentiviruses for luciferase (Con) or TSC2 (sh-TSC2), HepG2 cells were treated with BSA (−) or PA for 6 h and analysed by immunoblotting (n=3). (h–k) Five-month-oldSesn2−/−mice kept on HFD for 3 months were transduced once with adenoviruses expressing GFP (Con,n=5) or constitutive active AMPK (AMPKCA,n=6) (h,i) or were injected daily with vehicle (PBS,n=6) or AICAR (250 mg per kg body weight per day i.p.,n=5;j,k). After 10 days, livers were harvested, and protein phosphorylation and expression were examined (h,j) and quantified (i,k). All data are shown as the mean±s.e.m.Pvalues are from Student’st-test. Molecular weight markers are indicated in kDa. Figure 4: Sestrin2 controls ER homeostasis through the AMPK-mTORC1 axis. ( a – c ) HepG2 cells stably transduced with Sestrin2 shRNA (sh-Sesn2) were treated with PA for indicated hours ( a ) or 6 h ( b ). PBS (Con), AICAR (1 mM), Rapamycin (Rap, 100 nM), PP242 (1 μM), cycloheximide (CHX, 180 μM), BHA (100 μM) and NAC (10 mM) were applied 1 h before treating with PA. AICAR is an AMPK activator, PP242 is an mTOR inhibitor and CHX is a protein translation inhibitor. Protein phosphorylation and expression were examined ( a , b ) and quantified ( c ) ( n =3). P values were calculated between PA+PBS (Con) and indicated groups. ( d , e ) Sestrin2-silenced HepG2 cells were transduced with shRNA lentiviruses for luciferase (Con) or Raptor (sh-Raptor). After 48 h, cells were treated with BSA (−) or PA for 6 h and analysed by immunoblotting ( n =3). ( f , g ) At 48 h after infection with shRNA lentiviruses for luciferase (Con) or TSC2 (sh-TSC2), HepG2 cells were treated with BSA (−) or PA for 6 h and analysed by immunoblotting ( n =3). ( h – k ) Five-month-old Sesn2 −/− mice kept on HFD for 3 months were transduced once with adenoviruses expressing GFP (Con, n =5) or constitutive active AMPK (AMPK CA , n =6) ( h , i ) or were injected daily with vehicle (PBS, n =6) or AICAR (250 mg per kg body weight per day i.p., n =5; j , k ). After 10 days, livers were harvested, and protein phosphorylation and expression were examined ( h , j ) and quantified ( i , k ). All data are shown as the mean±s.e.m. P values are from Student’s t -test. Molecular weight markers are indicated in kDa. Full size image Sestrin2 is required to prevent liver damage during obesity As excessive ER stress can result in cell death [7] , [8] , we examined whether Sestrin2 is required for ensuring cell’s viability during ER stress insults. Upon prolonged SFA treatment for 16–24 h, Sestrin2-deficient HepG2 cells and mouse primary hepatocytes exhibited remarkably increased apoptotic cell death compared with control cells ( Supplementary Fig. 8a–d ), consistent with heightened ER stress level ( Supplementary Fig. 4a–d ). Sesn2 −/− mouse liver, upon Tm-induced ER stress, also exhibited more severe liver damage manifested by ectopic hepatocyte apoptosis and substantial elevation in serum alanine aminotransferase (ALT) levels compared with WT mouse liver ( Supplementary Fig. 8e–g ). More strikingly, HFD- or Lep ob -induced obesity, which by itself does not induce any liver damage in WT mice, provoked Sesn2 −/− mice to exhibit extensive hepatocyte death ( Fig. 5a,b ) and prominently elevated ALT levels ( Fig. 5c ), both of which were completely resolved by liver-specific reconstitution of Sestrin2 ( Fig. 5d–f ). TUDCA and salubrinal also effectively suppressed liver damage of obese or Tm-treated Sesn2 −/− mice ( Fig. 5g–i and Supplementary Fig. 7f,g ), suggesting that unresolved hepatic ER stress is the main cause of the liver damage observed. These data collectively highlight Sestrin2 as a critical hepatoprotective agent that prevents hepatocyte apoptosis and liver damage upon both acute and chronic ER stress. 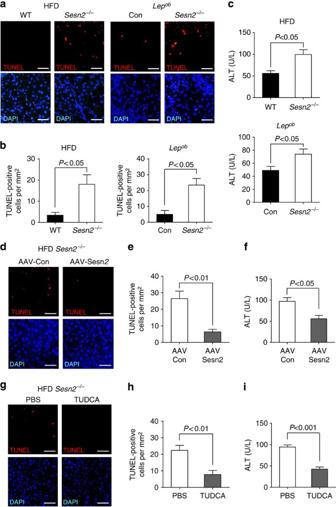Figure 5: Sestrin2 prevents liver damage during obesity. (a–c) Livers and sera were collected from 6-month-old WT (n=6) andSesn2−/−(n=5) mice kept on HFD for 4 months (HFD panels) or from 4-month-oldLepob/ob/Sesn2+/−(Con,n=4) andLepob/ob/Sesn2−/−(n=6) mice kept on LFD (Lepobpanels). Liver sections were subjected to TUNEL (red) and DAPI (blue) staining (a). TUNEL-positive cells were quantified (b). Serum ALT levels were quantified from indicated groups of mice (c). (d–f) Livers from obeseSesn2−/−mice transduced with AAV-Con (n=4) or AAV-Sesn2 (n=3) were subjected to TUNEL (red) and DAPI (blue) staining (d). TUNEL-positive cells in livers (e) and serum ALT levels (f) were quantified. (g–i) Five-month-oldSesn2−/−mice kept on HFD for 3 months were daily injected with vehicle (PBS,n=4) or TUDCA (500 mg per kg body weight per day i.p.,n=5). After 10 days of the treatment, mice were killed, and livers and sera were collected. Livers were subjected to TUNEL (red) and DAPI (blue) staining (g). TUNEL-positive cells in livers (h) and serum ALT levels (i) were quantified. Scale bars, 100 μm. All data are shown as the mean±s.e.m.Pvalues are from Student’st-test. Figure 5: Sestrin2 prevents liver damage during obesity. ( a – c ) Livers and sera were collected from 6-month-old WT ( n =6) and Sesn2 −/− ( n =5) mice kept on HFD for 4 months (HFD panels) or from 4-month-old Lep ob/ob / Sesn2 +/− (Con, n =4) and Lep ob/ob / Sesn2 −/− ( n =6) mice kept on LFD ( Lep ob panels). Liver sections were subjected to TUNEL (red) and DAPI (blue) staining ( a ). TUNEL-positive cells were quantified ( b ). Serum ALT levels were quantified from indicated groups of mice ( c ). ( d – f ) Livers from obese Sesn2 −/− mice transduced with AAV-Con ( n =4) or AAV-Sesn2 ( n =3) were subjected to TUNEL (red) and DAPI (blue) staining ( d ). TUNEL-positive cells in livers ( e ) and serum ALT levels ( f ) were quantified. ( g – i ) Five-month-old Sesn2 −/− mice kept on HFD for 3 months were daily injected with vehicle (PBS, n =4) or TUDCA (500 mg per kg body weight per day i.p., n =5). After 10 days of the treatment, mice were killed, and livers and sera were collected. Livers were subjected to TUNEL (red) and DAPI (blue) staining ( g ). TUNEL-positive cells in livers ( h ) and serum ALT levels ( i ) were quantified. Scale bars, 100 μm. All data are shown as the mean±s.e.m. P values are from Student’s t -test. Full size image Sestrin2 is an endogenous attenuator of steatohepatitis We found that dying hepatocytes in the liver of obese Sesn2 −/− mice were frequently associated with aggregation of dense-nucleated cells ( Supplementary Fig. 9a ), most of which were identified as F4/80-positive macrophages ( Supplementary Fig. 9b ). Some of the aggregated macrophages were proliferative as judged from positive BrdU staining ( Supplementary Fig. 9c ). As a result, the liver of obese Sesn2 −/− mice accumulated a highly increased number of macrophages ( Fig. 6a,b ), and these characteristics clearly imply the occurrence of active steatohepatitis. The steatohepatitis phenotype was completely suppressed by liver-specific Sestrin2 reconstitution ( Fig. 6c,d ), TUDCA administration ( Fig. 6e,f ) and AMPK reactivation ( Fig. 6g,h ). In addition, Sesn2 loss also aggravated Tm-induced steatohepatitis ( Supplementary Fig. 9d,e ). 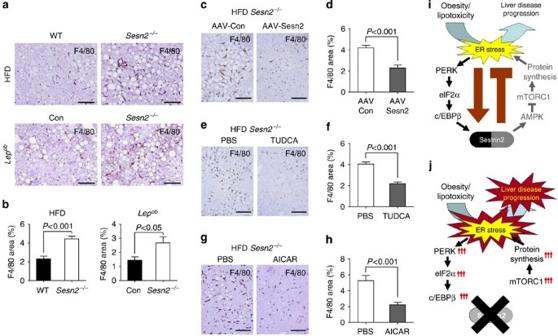Figure 6: Sestrin2 is an endogenous attenuator of steatohepatitis progression. (a,b) Livers from WT andSesn2−/−mice kept on HFD (HFD panels) orLepob/ob/Sesn2+/−(Con) andLepob/ob/Sesn2−/−mice kept on LFD (Lepobpanels) were subjected to anti-F4/80 staining to visualize macrophage infiltration (a). F4/80-positive areas were quantified (b). (c–h) Livers from obeseSesn2−/−mice transduced with AAV-Con (n=4) or AAV-Sesn2 (n=3) (c,d) or injected with PBS (n=4) or TUDCA (n=5) (e,f) or PBS (n=6) or AICAR (n=5) (g,h) were analysed with anti-F4/80 staining (c,e,g). F4/80-positive areas were quantified (d,f,h). Nuclei were visualized with haematoxylin (a,c,e,g). (i,j) Working model of how Sestrin2-mediated UPR attenuates NAFLD progression. In the WT liver, Sestrin2 is induced during obesity through the PERK–c/EBPβ pathway to attenuate protein translation and thereby relieve ER stress (i). InSesn2−/−liver, persistent mTORC1 activity elevates protein synthesis and subsequently aggravates ER stress, leading to facilitated NAFLD progression (j). Scale bars, 200 μm. All data are shown as the mean±s.e.m.Pvalues are from Student’st-test. Figure 6: Sestrin2 is an endogenous attenuator of steatohepatitis progression. ( a , b ) Livers from WT and Sesn2 −/− mice kept on HFD (HFD panels) or Lep ob/ob / Sesn2 +/− (Con) and Lep ob/ob / Sesn2 −/− mice kept on LFD ( Lep ob panels) were subjected to anti-F4/80 staining to visualize macrophage infiltration ( a ). F4/80-positive areas were quantified ( b ). ( c – h ) Livers from obese Sesn2 −/− mice transduced with AAV-Con ( n =4) or AAV-Sesn2 ( n =3) ( c , d ) or injected with PBS ( n =4) or TUDCA ( n =5) ( e , f ) or PBS ( n =6) or AICAR ( n =5) ( g , h ) were analysed with anti-F4/80 staining ( c , e , g ). F4/80-positive areas were quantified ( d , f , h ). Nuclei were visualized with haematoxylin ( a , c , e , g ). ( i , j ) Working model of how Sestrin2-mediated UPR attenuates NAFLD progression. In the WT liver, Sestrin2 is induced during obesity through the PERK–c/EBPβ pathway to attenuate protein translation and thereby relieve ER stress ( i ). In Sesn2 −/− liver, persistent mTORC1 activity elevates protein synthesis and subsequently aggravates ER stress, leading to facilitated NAFLD progression ( j ). Scale bars, 200 μm. All data are shown as the mean±s.e.m. P values are from Student’s t -test. Full size image Sestrin2 deficiency provokes liver fibrosis in obese mice Hepatocyte death and subsequent activation of liver inflammation can lead to activation of hepatic stellate cells (HSCs) that are known to secrete collagen. Although the liver from obese WT mice only displayed a few activated HSCs, visualized with alpha-smooth muscle actin (α-SMA) staining, the liver from obese Sesn2 −/− mice contained a substantially increased number of activated HSCs ( Supplementary Fig. 9f,g ). Consistent with this finding, there was a significant increase in collagen deposition in the liver from obese Sesn2 −/− mice ( Supplementary Fig. 9h,i ), validating the occurrence of liver fibrosis. Extensive fibrosis observed in the Lep ob/ob / Sesn2 −/− mouse liver was particularly striking because Lep ob/ob mutant mice were reported to be very resistant to liver fibrosis [3] . Taken together, these data collectively indicate that, during obesity, Sestrin2-mediated ER stress suppression is critical for preventing NASH-like liver pathologies including fibrosis ( Fig. 6i,j ). Sestrin2 regulates metabolism through ER stress suppression Persistent activation of ER stress signalling can provoke excessive fat accumulation and insulin resistance [14] , [15] . Tm-induced liver fat accumulation became more prominent and persistent upon Sestrin2 deficiency ( Supplementary Fig. 10a,b ). Although neither Tm nor Sestrin2 deficiency significantly increased the expression of genes responsible for hepatic lipogenesis ( Supplementary Fig. 10c ) as previously reported [12] , [22] , serum triglyceride level, which is usually decreased by Tm-induced ER stress [23] , was even further lowered by loss of Sesn2 ( Supplementary Fig. 10d ). The rapid reduction in the plasma lipid level upon ER stress reflects defective secretion of lipoproteins from hepatocytes [23] , [24] , which also causes acute hepatosteatosis. These results raise a possibility that Sestrin2 may control liver metabolism through regulating ER homeostasis. Indeed, increased hepatosteatosis and hepatic insulin resistance phenotypes of obese Sesn2 −/− mice ( Fig. 7a–d ) [12] , [25] were strongly suppressed by liver-specific reconstitution of Sestrin2 ( Fig. 7e–h ) or TUDCA administration ( Fig. 7i–l ), either of which can prevent hepatic ER stress. Thus, Sestrin2-mediated suppression of hepatic ER stress is not only required to prevent liver damage but also critical for proper regulation of lipid and glucose homeostasis. 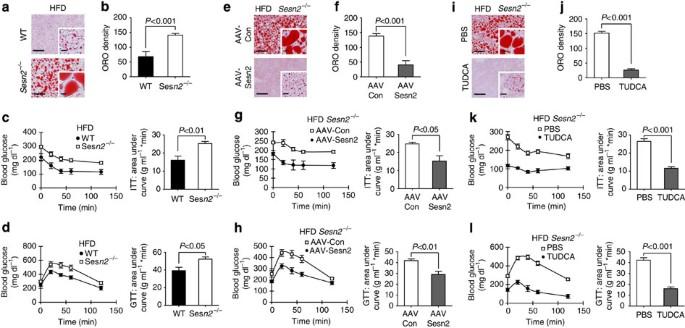Figure 7: Sestrin2 controls liver metabolism through regulating ER homeostasis. (a–d) Six-month-old WT andSesn2−/−mice were kept on HFD for 4 months. Livers were analysed with Oil Red O (ORO) staining (a). ORO densities were quantified (b) (n=4). Mice were tested for insulin resistance (ITT;c;n=8) and for glucose tolerance (GTT;d;n=8). Area-under-the-curve data for ITT (c) and GTT (d) were calculated. (e–h) Five-month-oldSesn2−/−mice kept on HFD for 3 months were transduced with AAV-Con (n=4) or AAV-Sesn2 (n=3). After 10 days, livers were harvested from the treated mice and analysed with ORO staining (e). ORO densities were quantified (f). Mice were tested for insulin resistance at 5 days (g) and for glucose tolerance at 7 days (h) after AAV transduction. Area-under-the-curve data for ITT (g) and GTT (h) were calculated. (i–l) Five-month-oldSesn2−/−mice kept on HFD for 3 months were daily injected with vehicle (PBS,n=4) or TUDCA (500 mg per kg body weight per day i.p.,n=5). After 10 days of treatment, livers were harvested from the treated mice and analysed with ORO staining (i). ORO densities were quantified (j). Mice were tested for insulin resistance at 5 days (k) and for glucose tolerance at 7 days (l) after initiation of TUDCA treatment. Area-under-the-curve data for ITT (k) and GTT (l) were calculated. Scale bars, 200 μm; 10 μm (insets). All data are shown as the mean±s.e.m.Pvalues are from Student’st-test. Figure 7: Sestrin2 controls liver metabolism through regulating ER homeostasis. ( a – d ) Six-month-old WT and Sesn2 −/− mice were kept on HFD for 4 months. Livers were analysed with Oil Red O (ORO) staining ( a ). ORO densities were quantified ( b ) ( n =4). Mice were tested for insulin resistance (ITT; c ; n =8) and for glucose tolerance (GTT; d ; n =8). Area-under-the-curve data for ITT ( c ) and GTT ( d ) were calculated. ( e – h ) Five-month-old Sesn2 −/− mice kept on HFD for 3 months were transduced with AAV-Con ( n =4) or AAV-Sesn2 ( n =3). After 10 days, livers were harvested from the treated mice and analysed with ORO staining ( e ). ORO densities were quantified ( f ). Mice were tested for insulin resistance at 5 days ( g ) and for glucose tolerance at 7 days ( h ) after AAV transduction. Area-under-the-curve data for ITT ( g ) and GTT ( h ) were calculated. ( i – l ) Five-month-old Sesn2 −/− mice kept on HFD for 3 months were daily injected with vehicle (PBS, n =4) or TUDCA (500 mg per kg body weight per day i.p., n =5). After 10 days of treatment, livers were harvested from the treated mice and analysed with ORO staining ( i ). ORO densities were quantified ( j ). Mice were tested for insulin resistance at 5 days ( k ) and for glucose tolerance at 7 days ( l ) after initiation of TUDCA treatment. Area-under-the-curve data for ITT ( k ) and GTT ( l ) were calculated. Scale bars, 200 μm; 10 μm (insets). All data are shown as the mean±s.e.m. P values are from Student’s t -test. Full size image Although Sestrin2 was originally identified as a protein inducible upon DNA damage and oxidative stress [26] , these stress insults turned out to be not responsible for Sestrin2 upregulation during obesity. Rather, disruption of ER homeostasis was the critical event responsible for obesity-induced Sestrin2 expression. An ER stress sensor PERK and its downstream transcription factor c/EBPβ play essential roles in Sestrin2 upregulation upon nutritionally or chemically induced ER stress. Other signalling mediators of ER stress, such as IRE1, ATF6, ATF4, CHOP and JNK, appeared not to be significantly involved in this process. As Sestrin2 is the only Sestrin-family protein inducible upon obesity or ER stress, loss of Sesn2 was not compensated by the presence of Sestrin1 or Sestrin3. This allowed us to investigate the physiological functions of Sestrin2 in the context of ER stress using Sestrin2-deficient cells and mice. Sestrin2-deficient cells cannot cease protein translation upon prolonged ER stress insults even though they exhibit prominently elevated PERK-eIF2α signalling activities. This finding was particularly striking to us because it has been formerly believed that ER stress-induced translation arrest is solely and directly mediated by PERK-dependent phosphorylation of eIF2α (ref. 6 ). However, according to our results, Sestrin2-mediated mTORC1 regulation can be another important mechanism that can suppress protein translation during chronic ER stress. As Sestrin2-deficient cells lack this mechanism, they exhibited excessive ER stress that induces activation of the PERK-eIF2α signalling as well as the other branches of ER stress signalling. Increased ER stress observed in Sestrin2-deficient cells was suppressible by genetic or pharmacological inhibition of mTORC1. Therefore, Sestrin2-mediated mTORC1 regulation is an important UPR mechanism downstream of the PERK–eIF2α–c/EBPβ signalling that prevents excessive accumulation of unfolded proteins and aggravation of ER stress ( Fig. 6i,j ). Recent reports have shown that deregulation of mTORC1 or protein translation can promote accumulation of unfolded and misfolded proteins, thereby further sensitizing cells to ER stress insults [27] , [28] , [29] . Consistent with these, Sestrin2-deficient hepatocytes were hypersusceptible to ER stress-induced cell death, and Sesn2 −/− mice were prone to develop ER stress-induced liver pathologies associated with hepatocyte death. The liver pathologies were suppressed by either AICAR or TUDCA administration, suggesting that defective AMPK-mTORC1 regulation and subsequent exacerbation of ER stress are the causes of these pathologies. In summary, we have described a role for Sestrin2 as the critical component of hepatic UPR that mediates ER stress-induced suppression of protein synthesis. Sestrin2-mediated UPR mechanism is important for suppression of obesity-associated NAFLD pathologies including liver damage and steatohepatitis as well as fat accumulation and insulin resistance. Sestrin2’s protective role against ER stress may be also important in other non-hepatic tissues that may experience increased levels of ER stress during obesity. Considering that unresolved ER stress is a possible pathogenetic cause of diverse diseases including cancer, neurodegeneration, type 1/2 diabetes and atherosclerosis [9] and that obesity increases incidences of these degenerative diseases [30] , it would be much of interest to investigate possible protective roles of Sestrin2 against progression of these degenerative diseases beyond the scope of liver pathologies. Antibodies and reagents Antibodies against Sestrin1 and Sestrin2 were generated from bacterially expressed recombinant proteins as described [12] . Antibodies against phospho-PERK (Cell Signaling, Santa Cruz), PERK (Cell Signaling, Santa Cruz), ATF4 (Santa Cruz), ATF6 (Santa Cruz), c/EBPβ (Santa Cruz), RNA polymerase II (Santa Cruz), SERCA2 (Santa Cruz), phospho-S6 kinase (Cell Signaling, Santa Cruz), S6K (Santa Cruz), phospho-AMPKα (Santa Cruz), AMPKα (Santa Cruz), CHOP (Cell Signaling, Santa Cruz), IRE1α (Santa Cruz), heavy chain-binding protein (BiP; Cell Signaling), protein disulphide isomerase (Cell Signaling), phospho-JNK (Cell Signaling), JNK (BD Biosciences), p53 (Santa Cruz), phospho-c-Jun (Santa Cruz), c-Jun (Santa Cruz), phospho-S6 (Cell Signaling), S6 (Cell Signaling), phospho-eIF4E-binding protein (Cell Signaling), 4E-BP (Cell Signaling), phospho-eIF2α (Cell Signaling), eIF2α (Santa Cruz), Raptor (Cell Signaling), TSC2/tuberin (Santa Cruz), Sestrin2 (Proteintech), Sestrin3 (Abcam), F4/80 (Invitrogen), α-SMA (Abcam), Actin (DSHB), puromycin (DSHB) and Tubulin (Sigma) were used as primary antibodies. Horseradish peroxidase (HRP)-conjugated secondary antibodies (Bio-Rad), biotin-conjugated secondary antibodies (BD Biosciences), streptavidin-HRP (BD Biosciences) and Alexa Flour-conjugated secondary antibodies (Invitrogen) were used for immunoblotting and immunostaining procedures. Fatty acid free and low endotoxin bovine serum albumin (BSA), PA, stearic acid, oleic acid, docosahexaenoic acid, Tm, thapsigargin, insulin, glucose, Oil Red O, butylated hydroxyanisole and N-acetyl cysteine were purchased from Sigma. Cycloheximide was from Amresco and PP242 was from Chemdea. TUDCA was purchased from EMD Millipore. SP600125, rapamycin and AICAR were purchased from LC Labs. Salubrinal was purchased from Calbiochem. Cell culture HepG2 cells (gift from Dr Saltiel) were maintained in Dulbecco’s modified Eagle’s medium (DMEM, Invitrogen) containing 10% fetal bovine serum (fetal bovine serum, Sigma), 50 U ml −1 penicillin and 50 mg ml −1 streptomycin. De-lipidated low-endotoxin BSA was loaded with indicated fatty acids and applied to cultured cells as described [31] . Mice and diets WT, Sesn2 −/− and Lep ob/ob mice are in the C57BL/6 background as described [12] . Male mice of indicated age were used for the study. Mice were maintained in filter-topped cages and were given free access to autoclaved regular chow diet (low-fat diet) or HFD (composed of 59% fat, 15% protein and 26% carbohydrates based on caloric content; Bio-Serv) and water at the University of Michigan (UM) according to the NIH and institutional guidelines. All animal studies were overseen by the University Committee on Use and Care of Animals at UM. Lentiviruses The lentiviral plasmids for sh-Sestrin2 (ref. 10 ), sh-p53 (ref. 32 ), sh-c/EBPβ [33] , sh-Raptor and sh-TSC2 (ref. 12 ) were previously described. Lentiviral plasmids for sh-PERK (TRCN0000001401 and TRCN0000001399), sh-ATF6 (TRCN0000017853 and TRCN0000017855), sh-CHOP (TRCN0000007264) and sh-ATF4 (TRCN0000013575) were purchased from Open Biosystems (Huntsville, AL). Lentiviral IRE1α DN construct was obtained from Addgene (Cambridge, MA). Lentiviruses were generated in the Vector Core facility at the UM. Adenoviruses Adenoviruses expressing AMPK CA (Ad-AMPK CA ) were purchased from Eton Biosciences. Adenoviruses expressing the 2b isoform of SERCA2 (Ad-SERCA2b) were gifts from Dr Hotamisligil [15] . Adenoviruses expressing c/EBPβ and sh-c/EBPβ were gifts from Dr Lin [34] . Control adenoviruses were supplied by the UM Vector Core. Adeno-associated viruses (AAVs) for green fluorescent protein (GFP; AAV-Con) and Sestrin2 (AAV-Sesn2) were gifts from Dr Pura Munoz (UPF, Spain). The viruses were amplified in the UM Vector Core. For hepatic gene transfer, 10 9 plaque-forming units of viruses were injected into mice through their tail vein. Immunoblotting Cells or tissues were lysed in RIPA buffer (50 mM Tris-Cl, pH 7.4, 150 mM NaCl, 1% sodium deoxycholate, 1% NP-40; 0.1% SDS) or cell lysis buffer (20 mM Tris-Cl, pH 7.5, 150 mM NaCl, 1 mM EDTA, 1 mM EGTA, 2.5 mM sodium pyrophosphate, 1 mM β-glycerophosphate, 1 mM Na 3 VO 4 , 1% Triton-X-100) containing protease inhibitor cocktail (Roche). After being clarified with centrifugation, lysates were boiled in SDS sample buffer, separated by SDS–PAGE, transferred to polyvinylidene difluoride membranes and probed with the indicated antibodies. Primary antibody dilution factors were 1:200 (all Santa Cruz antibodies), 1:100 (anti-puromycin antibody) or 1:1,000 (all other antibodies). After incubation with secondary antibodies conjugated with HRP (1:2,000), chemiluminescence was detected and quantified using LAS4000 (GE) system. Full-sized scans of all western blots are provided in Supplementary Fig. 11 . Quantitative reverse transcriptase/real-time PCR (qRT–PCR) Total RNA was extracted from tissues or cells using Trizol reagent (Invitrogen), and cDNA was made using MMLV-RT (Promega) and random hexamers (Invitrogen). Quantitative PCR was performed in a Real-Time PCR detection system (Applied Biosystems) with iQ SYBR Green Supermix (Bio-Rad) and relevant primers. Relative mRNA expression was calculated from the comparative threshold cycle ( C t ) values relative to Cyclophilin A (CypA). Primers for human Sestrin1–3 (ref. 35 ), human CypA [36] , human XBP1 (ref. 37 ), mouse XBP1 (ref. 38 ), active spliced form of mouse XBP1 (ref. 38 ) and human XBP1 (ref. 39 ), mouse BiP [40] , mouse ER degradation-enhancing alpha-mannosidase-like 1 (ref. 40 ), mouse ER oxidoreductin-1α (ref. 40 ), human CHOP [36] , mouse CHOP [40] , mouse protein disulphide isomerase [41] , mouse ER-localized DnaJ homologue 4 (ref. 41 ), mouse HMG-CoA reductase [42] , mouse sterol regulatory element-binding transcription factor 1 (ref. 42 ), mouse Srebf2 (ref. 42 ), mouse fatty acid synthase [43] , mouse acetyl-CoA carboxylase alpha (Acaca) [43] , mouse Acacb [43] , mouse β-Actin [44] and mouse CypA [12] were designed as described. The ratio of spliced (XBP1-s) to unspliced (XBP1-u) XBP1 levels was determined using semi-quantitative RT–PCR; PCR products of XBP1-s and XBP1-u were separated using electrophoresis on a 2.5% agarose gel and visualized with ethidium bromide staining. Percent of XBP1 splicing was quantified using ImageJ (NIH). Histology Liver tissues were fixed in 10% buffered formalin, embedded in paraffin and stained with haematoxylin and eosin. To visualize collagen fibres, liver sections were stained with saturated picric acid containing 0.5% Sirius Red (Sigma). The sections were washed with distilled water, dehydrated, mounted and analysed with light microscopy. For immunostaining of BiP, p-PERK and F4/80, paraffin-embedded liver sections were incubated with corresponding primary antibodies (1:200, 1:50 and 1:100, respectively), followed by incubation with biotin-conjugated secondary antibodies (1:200) and streptavidin-HRP (1:300). The HRP activity was visualized with diaminobenzidine staining. Haematoxylin counterstaining was applied to visualize nuclei. For α-SMA staining, liver sections were incubated with anti-α-SMA antibody (1:100), followed by incubation with Alexa Flour 594-conjugated secondary antibody (1:250) and counterstaining with 4',6-diamidino-2-phenylindole (DAPI; Invitrogen). TdT-mediated dUTP nick end labelling (TUNEL) assay was performed using In Situ Cell Death Detection Kit-TMR-Red (Roche). Samples were analysed under an epifluorescence-equipped light microscope (Olympus). Glucose and insulin tolerance tests (GTT and ITT) For GTT and ITT, mice that were made to fast for 6 h were injected with glucose (1 g per kg body weight intraperitoneally (i.p.)) or insulin (0.65 U per kg body weight i.p.). Blood glucose was instantly measured at 0, 20, 40, 60 and 120 min after glucose or insulin injection using OneTouch Ultra glucose meter. Oil Red O staining Optimum cutting temperature compound (OCT)-embedded frozen liver sections were allowed to air dry and were rinsed with 60% isopropanol, followed by staining with fresh 0.5% Oil Red O solution for 15 min. After staining, the slides were rinsed with 60% isopropanol, washed with distilled water, mounted and analysed under light microscope (Olympus). Serum ALT assay Serum ALT levels were measured with an ALT activity assay kit (Sigma) according to the manufacturer’s instructions. ROS detection Intracellular level of ROS was measured using ROS indicator chloromethyl-2′,7′-dichlorodihydrofluorescein diacetate (CM-H 2 DCFDA, Invitrogen). Cells were treated with 5 μM CM-H 2 DCFDA for 30 min at 37 °C in the dark and washed in phosphate-buffered saline, followed by observation under an epifluorescence-equipped microscope (Olympus). Dihydroxyethidium staining of liver tissues was carried out as described using freshly frozen sections [45] . Primary cell culture Primary mouse hepatocytes were isolated from livers of 2-month-old lean WT or Sesn2 −/− mice, as described [46] . Immunocytochemistry For c/EBPβ staining, HepG2 cells were fixed with methanol and incubated with anti-c/EBPβ antibody (1:100), followed by incubation with Alexa Fluor 594-conjugated secondary antibody (1:500) and counterstaining with DAPI (Invitrogen). Samples were analysed under an epifluorescence-equipped light microscope (Olympus). Measurement of protein synthesis To label newly synthesized proteins with L-azidohomoalanine (AHA) in cultured cells, cells were incubated with 25 μM AHA (Invitrogen) in methionine- and cysteine-free DMEM (Invitrogen) for 3 h in the presence of 10% fetal bovine serum and antibiotics. AHA-incorporated proteins were labelled with biotin using Click-iT Biotin Protein Analysis Detection Kit (Invitrogen). The biotin-labelled proteins were assayed by immunoblotting. To label newly synthesized proteins with AHA in the mouse liver, mice were injected with 13 mg per kg body weight AHA (i.p.). After 15 min, the liver was harvested and analysed using Click-IT immunoblotting. To label nascent peptides with puromycin, cultured cells were incubated with 1 μM puromycin (Calbiochem) in normal culture medium, and mice were injected with 0.04 mmol per kg body weight puromycin (i.p.). After 30 min, cells and livers were harvested and puromycin-labelled proteins were detected using anti-puromycin immunoblotting. Luciferase assay The luciferase-based Sesn2 reporter constructs and c/EBP DN plasmid were described previously [47] . HepG2 cells were transfected with Sesn2 -luciferase constructs and renilla luciferase expression vector (pTK-RL) using Lipofectamine 2000 (Invitrogen). After 48 h, cells were treated with BSA or PA for 9 h. Luciferase activity was analysed using Dual-Luciferase reporter assay kit (Promega). Chromatin immunoprecipitation (ChIP) HepG2 cells were treated with BSA or PA for 9 h and fixed with 1% paraformaldehyde for 10 min at room temperature. ChIP assays were performed using the EZ-ChIP Kit (EMD Millipore) according to the manufacturer’s instructions. Chromatin extracts were immunoprecipitated with anti-c/EBPβ or anti-RNA polymerase II antibodies. Protein-associated DNA was analysed with quantitative PCR using the following primers targeting sequences between −278 and +13 bps from the transcription start site of the Sesn2 gene: 5′-TCCCTTTTCATCACGCAACC-3′ and 5′-CTCTGACACCAGCAGTTCAGC-3′. Statistical analysis Statistical significance of differences between two groups was calculated by a two-tailed Student’s t -test. P values equal to or above 0.05 were considered not statistically significant. How to cite this article: Park, H.-W. et al. Hepatoprotective role of Sestrin2 against chronic ER stress. Nat. Commun. 5:4233 doi: 10.1038/ncomms5233 (2014).